Magnetic control of transverse electric polarization in BiFeO3 Numerous attempts have been made to realize crossed coupling between ferroelectricity and magnetism in multiferroic materials at room temperature. BiFeO 3 is the most extensively studied multiferroic material that shows multiferroicity at temperatures significantly above room temperature. Here we present high-field experiments on high-quality mono-domain BiFeO 3 crystals reveal substantial electric polarization orthogonal to the widely recognized one along the trigonal c axis. This novel polarization appears to couple with the domains of the cycloidal spin order and, hence, can be controlled using magnetic fields. The transverse polarization shows the non-volatile memory effect at least up to 300 K. Magnetism and ferroelectricity are two representative subjects in condensed matter physics. The quest to understand their fundamentals has clarified how various materials can exhibit such properties, resulting in the development of various indispensable devises. However, these properties of solids are usually mutually exclusive in materials [1] . Although some exceptional materials, exhibiting both properties, have been recognized as ferroelectric magnets for over 40 years, the rich physics attributed to their cross-correlation had long remained unknown. The recent discovery of magnetic control of the electric polarization in manganite [2] has attracted significant attention in pure and applied science. The following large number of studies revealed three major microscopic scenarios to induce the electric polarization by the spin system [3] : spin current [4] , [5] , [6] , exchange striction [7] , [8] and spin-dependent p – d hybridization mechanisms [9] , [10] , [11] . The first scenario, called spin–current or inverse Dzyaloshinskii–Moriya mechanism, predicted the emergence of the electric polarization ( P ) expressed by the vector spin chirality of the adjacent spins ( S i , j ) and the unit vector connecting these sites ( e ij ) as P ∝ e ij × ( S i × S j ). This simple expression supported the excavation of multiferroic materials in which electric polarization can be controlled by external magnetic fields. The vector spin chirality in localized spin system is usually caused by the frustration between spin interactions. Inevitably, the magnetic ordering temperature is low in the frustrated spin systems. A large number of efforts have been devoted to realize high-temperature multiferroic and/or magnetoelectric (ME) materials [12] , [13] , [14] , [15] , aiming to apply multiferroics to practical devices such as low-power-consumption memory devices. Although some of them exhibit significant ME effects at room temperature [13] , [14] , [15] , the electric polarization is absent or negligibly small at zero magnetic field and, hence, external magnetic fields are required to control the dielectric state. BiFeO 3 is unique, because it exhibits substantial multiferroicity well above room temperature [16] . It belongs to the trigonal R 3 c space group ( Fig. 1 ) below ~1,100 K, owing to the displacement of ions along and normal to the ‹111› direction of the perovskite cubic unit ( c axis of the trigonal cell) and the rotation of the ions around the same axis. Spontaneous polarization emerges along this axis with the magnitude exceeding 400,000 μ C m −2 (ref. 17 ), which is superior to those of typical ferroelectric compounds such as BaTiO 3 . As BiFeO 3 shows eight-fold degeneracy in the directions of the trigonal c axis, its actual crystals often contain multiple crystallographic domains. 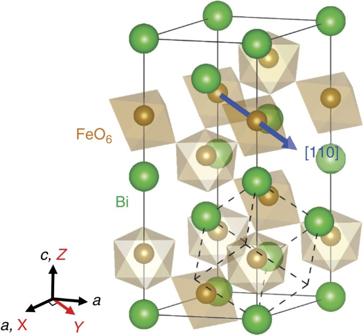Figure 1: Schematic crystal structure of BiFeO3. Thick blue arrow represents a direction of a spin modulation vector. Dashed lines represent the pseudo-cubic unit in the perovskite structure.X,YandZdenote Cartesian coordinates. Figure 1: Schematic crystal structure of BiFeO 3 . Thick blue arrow represents a direction of a spin modulation vector. Dashed lines represent the pseudo-cubic unit in the perovskite structure. X , Y and Z denote Cartesian coordinates. Full size image The spins of Fe 3+ ions form a cycloidal order with the propagation vector pointing ‹110› direction of the trigonal lattice below ~640 K [18] , [19] , [20] . Such a non-collinear state can be explained by the Ginzburg–Landau theory, including the ME coupling term [21] , or equivalently by the spin Hamiltonian, including Dzyaloshinskii–Moriya vectors normal to the c axis [22] , [23] . According to the spin–current mechanism, this cycloidal spin order involves P along the c axis. This magnetically induced component of P can be removed at the transition from the cycloidal to the canted-antiferromagnetic state induced by a high magnetic field [24] , [25] , and indeed observed by Popov et al. [24] . Quantitative evaluation of the ME effect can be done only through the experiments on mono-domain crystals, otherwise the crystallographic domain boundaries, which are known to be conductive [26] , deteriorate the intrinsic signal. Recent high-field experiments on the mono-domain crystals showed the change in P at the transition to be ~210±30 μ C m −2 below 400 K as a projected value on the cubic principal axis [27] . Details of the ME tensor remain open albeit indispensable to understand the multiferroicity of this material. In particular, we have to pay attention to the threefold degeneracy in the choice of the magnetic propagation vector that should affect the ME effects observed at low fields [28] . In the present study, we performed experiments along the trigonal coordinates to obtain a fundamental understanding of the ME effects in BiFeO 3 . Recently developed high-quality BiFeO 3 single crystals grown using the laser-diode heating floating-zone method [29] enabled these experiments. The results unexpectedly reveal the transverse (normal to the cycloidal spin rotation plane) component of the electric polarization >800 μ C m −2 , which is controllable using magnetic fields. This novel component cannot be understood by the spin–current mechanism. However, on a bond with lower symmetry, the anti-symmetric pair of the adjacent spins can couple to P in a generic formula P α ∝ ∑ β d αβ ( S i × S j ) β , where d is a tensor and non-zero components of it are determined by a local symmetry of the bonds [30] , [31] . In fact, all the tensor components of d are allowed on nearest-neighbour bonds in BiFeO 3 , which induce the coupling between the transverse component of the electric polarization and cycloidal spin structure. As a result, we can reasonably reproduce the novel transverse component, which is confined to the magnetic domains and, hence, is easily controlled using a moderately high magnetic field even at 300 K. Further, BiFeO 3 shows the irreversible ME effect up to 300 K, indicating its potential application in non-volatile memory devices. 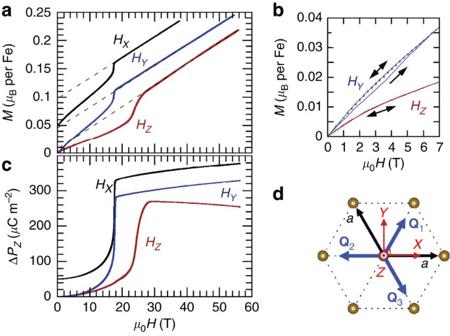Figure 2: Magnetic-field dependence of magnetization and electric polarization along theZaxis. (a) Magnetization curves for BiFeO3measured at 4.2 K forHapplied alongX(black),Y(blue), andZ(red) directions. The trace forHXwas vertically offset by 0.05μBper Fe for clarity. (b) Magnetization curves measured at 4.2 K up to 7 T. Thin lines and solid symbols represent data measured during first and second field scans, respectively. (c) Magnetic-field-induced changes in polarization measured alongZdirection (ΔPZ) for fields applied alongX,YandZdirections at 4.2 K. The data forHXwas vertically offset by 50μC m−2for clarity. (d) Schematic drawing of Cartesian coordinatesX,YandZ. Thick blue arrows represent direction of modulation vectors forQ1,Q2andQ3magnetic domains. Magnetization and the longitudinal electric polarization Figure 2a shows the magnetization ( M ) curves for BiFeO 3 . Most of the data were measured at 4.2 K, unless otherwise stated. Magnetic fields ( H ) were applied along the a axis, normal to the ca plane, and along the c axis, which are defined as the X , Y and Z directions, respectively ( Figs 1 and 2d ). For the H applied along the X direction, the M first slowly increased and then steeply increased at ~18 T. It then varied almost linearly with increasing H (black line). Linearly extrapolating the high-field M – H curve (dashed black line) gave a finite intercept of 0.048±0.002 μ B per Fe at the zero-field, which is consistent with the emergence of the high-field canted antiferromagnetic phase [25] . The H applied along the Y direction (blue line) exhibited a trace almost identical to that of the H applied along the X direction. The difference between the blue and black traces is barely distinguishable in Fig. 2a . The M for H || Z , on the other hand, gradually increased in the low field, steeply increased with increasing H between 22 and 26 T, and then varied linearly with increasing H up to 56 T. Extrapolating the M – H curve from the high-field phase to the zero-field indicated ferromagnetic components of 0.009±0.002 μ B per Fe, significantly lower than the trigonal plane ones, suggesting that the ferromagnetic moment was mostly confined to the trigonal plane. Figure 2: Magnetic-field dependence of magnetization and electric polarization along the Z axis. ( a ) Magnetization curves for BiFeO 3 measured at 4.2 K for H applied along X (black), Y (blue), and Z (red) directions. The trace for H X was vertically offset by 0.05 μ B per Fe for clarity. ( b ) Magnetization curves measured at 4.2 K up to 7 T. Thin lines and solid symbols represent data measured during first and second field scans, respectively. ( c ) Magnetic-field-induced changes in polarization measured along Z direction (Δ P Z ) for fields applied along X , Y and Z directions at 4.2 K. The data for H X was vertically offset by 50 μ C m −2 for clarity. ( d ) Schematic drawing of Cartesian coordinates X , Y and Z . Thick blue arrows represent direction of modulation vectors for Q 1 , Q 2 and Q 3 magnetic domains. Full size image Careful observation of the magnetization curve revealed hysteresis in the low-field region. Figure 2b shows the steady-field magnetization with increasing H to 7 T. The M – H curve for the H applied along the Y direction was hysteretic, as shown by the thin blue line. The M – H curve for the second field sweep coincided with the upper trace without showing hysteresis (solid blue symbols). The M – H curve for the H applied along the X direction (not shown) showed similar hysteretic behaviour. The M – H curve for the H applied along the Z direction, on the other hand, showed a reversible profile even for the first sweep (thin red line). We interpreted these hysteretic behaviours as the re-orientation of the magnetic domains in BiFeO 3 . Figure 2c shows the magnetic-field-induced change in the P along the Z direction (Δ P Z ). The effects of the H applied along the X and Y directions are almost identical. The difference between the blue and black traces is barely identifiable. The P Z first gradually increased and then steeply increased at the magnetic transition with increasing H . The P Z continuously changed above the transition field. The H applied along the Z direction also caused P Z to first gradually increase then steeply increased at the transition. The low-order ME effect above the transition field showed the opposite sign to that of the in-plane fields. Although we could not determine the sign of the Δ P Z with respect to the non-centrosymmetric crystal, the sign of the polarity relative to those of the different field directions is meaningful, because we changed the field direction while holding the wiring. 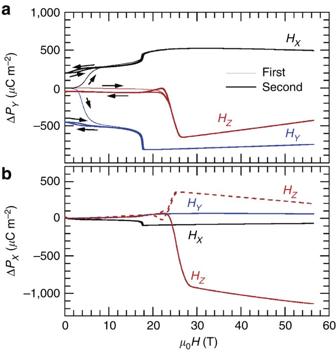Figure 3: Magnetic-field dependence of electric polarization along theXandYaxis. (a) Magnetic field dependence ofPYforHapplied alongX(black),Y(blue) andZ(red) directions. Thin and thick lines represent traces during first and second field scans, respectively. (b) Field-induced changes inPXforHapplied along all three directions. Dashed red line showsPX–HZcurve measured for a different piece of BiFeO3crystal. Magnetic control of the transverse electric polarization Figure 3a shows the change in the transverse component, P Y , for the H applied along the X , Y and Z directions. The thin black line shows that P Y steeply changed in the first trace for the H || X sweep at μ 0 H ≤7 T. Here, μ 0 is the space permeability. P Y then further increased ~100 μ C m −2 at the transition field and moderately changed with increasing H up to 56 T. P Y followed almost the same trace down to 10 T when the magnetic field was decreased, but did not significantly change in μ 0 H ≤7 T. The second sweep (thick black line) traced the profile of the previous down-sweep without showing any prominent hysteresis. Applying H Y also produced an irreversible P – H curve but in the opposite direction (thin blue line), while μ 0 H Y ≤7 T during the virgin scan. Further, Δ P Y at the transition field also showed the opposite sign from that for H || X and showed an almost linear ME effect with increasing H to the highest field. The P – H curve for H Z , on the other hand, showed marginal hysteresis for μ 0 H <20 T, steeply increased when μ 0 H ~26 T and then showed the linear ME effect. The observed Δ P Y amounted to 500–800 μ C m −2 and dominated the widely recognized P Z component caused by the cycloidal spin order ( Fig. 1c ). Figure 3: Magnetic-field dependence of electric polarization along the X and Y axis. ( a ) Magnetic field dependence of P Y for H applied along X (black), Y (blue) and Z (red) directions. Thin and thick lines represent traces during first and second field scans, respectively. ( b ) Field-induced changes in P X for H applied along all three directions. Dashed red line shows P X – H Z curve measured for a different piece of BiFeO 3 crystal. Full size image Figure 3b shows the H dependence of P X . The field-induced change in P X for H X and H Y is much smaller than those in P Y for the same, which remarkably contrasts with the almost isotropic magnetic properties observed in the magnetization measurements. Contrary to the small change in P X when the in-plane fields were applied, P X considerably changed only when H Z was applied. The solid red line in Fig. 3b shows that the Δ P X amounted to 800 μ C m −2 at the transition field and then showed the linear ME effect when the field was higher. This considerable change, however, was less reproducible. The dashed red line represents the P X – H Z profile measured for another piece of BiFeO 3 crystal. The change measured at the transition became much smaller and showed the opposite sign of the previous one, whereas the high-field phase showed a similar linear ME effect in the same sign. The origin of the prominent transverse polarization could be anti-symmetric spin pair-dependent electric polarization P α ∝ ∑ β d αβ ( S i × S j ) β , where d αβ is a coupling between spin and electric polarization [30] , [31] . For example, the cycloidal screw state with Q 2 have finite ( S i × S i + x ) Y [( S i × S i + y ) Y ] on bonds along ‹100› (‹010›) on a pseudo-cubic unit cell ( Supplementary Fig. 1 ), which produces P Y ∝ d YY [( S i × S i + x ) Y −( S i × S i + y ) Y ] in addition to the conventional term P Z ∝ d ZY [( S i × S i + x ) Y −( S i × S i + y ) Y ] due to the spin current mechanism. From the observed values of Δ P and the reported cycloidal spin structure [20] , the magnitudes of the coupling are estimated to be | d YY |=6.4 × 10 −32 C m and | d ZY |=4.5 × 10 −32 C m as described in Supplementary Note 1 . The results indicate that the coupling of P Y is larger than that of P Z . Owing to the symmetry of the crystal, the cycloidal screw states with Q 1 , Q 2 and Q 3 modulations can produce in-plane components of electric polarization ( P T ) normal to the spin rotation plane, which is spanned by the c axis and the spin modulation vector for each cycloidal domain ( Fig. 4a,b ). Applying magnetic fields is expected to favour the domains showing the spin rotation plane normal to the field. For example, applying H Y stabilizes the Q 2 domain as illustrated in Fig. 4a . Here, P X =0 and P Y = P T ( Fig. 4a ). Applying H X , on the other hand, favours the Q 1 and Q 3 domains; hence, P X ~0 if the BiFeO 3 contains the same number of each domain, while P Y =− P T /2 regardless of the number of each domain ( Fig. 4b ). In this scenario, P X becomes small when the field is applied along the X or Y directions, as was experimentally observed, whereas it can become large when the field is applied at intermediate angles within the X – Y plane. The response to applying H Z would be highly sensitive to possible field misalignment, as slight tilting towards a certain in-plane direction would determine the magnetic domains, that is, magnitude and direction of the P T , which are both consistent with the results shown in Fig. 3b . 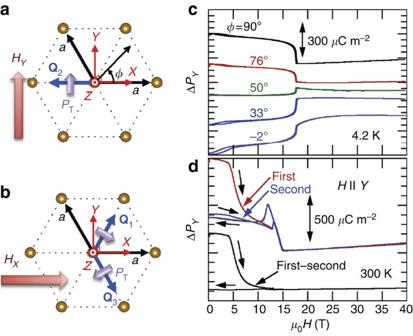Figure 4: Magnetic-field dependence of electric polarization along theYaxis at various field direction and at temperature of 300 K. Schematic drawings of magnetic field dependence of the magnetic domains for (a)H||Yand (b)H||X. Short violet arrows represent direction of transverse electric polarization vectors (PT) forQ1,Q2andQ3magnetic domains. (c) Magnetic field dependence ofPYmeasured at various angles in range −2°≤φ≤90°. (d)PY–HYcurve measured at 300 K. Red and blue lines represent traces for first and second field scans, respectively. Black line shows difference between them. Data inFig. 4c,dwere vertically offset for clarity. Figure 4: Magnetic-field dependence of electric polarization along the Y axis at various field direction and at temperature of 300 K. Schematic drawings of magnetic field dependence of the magnetic domains for ( a ) H || Y and ( b ) H || X . Short violet arrows represent direction of transverse electric polarization vectors ( P T ) for Q 1 , Q 2 and Q 3 magnetic domains. ( c ) Magnetic field dependence of P Y measured at various angles in range −2°≤ φ ≤90°. ( d ) P Y – H Y curve measured at 300 K. Red and blue lines represent traces for first and second field scans, respectively. Black line shows difference between them. Data in Fig. 4c,d were vertically offset for clarity. Full size image To investigate these hypotheses, we studied the field dependence of P Y by changing the field direction within the X – Y plane. Figure 4c shows P Y plotted as functions of the H measured at various azimuthal angles, φ , from the X direction. The change in P Y at the transition field changed its sign between 50° and 76° with increasing the φ , which is consistent with the expectation from our simple domain model in which the most stable domain changed from Q 3 ( P Y =− P T /2) to Q 2 ( P Y = P T ) at φ =60°. The results so far suggest that a large transverse polarization was coupled with magnetic domains of BiFeO 3 . The irreversible magnetic and dielectric behaviour for μ 0 H <10 T suggests that the re-orientation of the magnetic domains was preserved even after the H was removed. To check whether the memory effect could be observed even at room temperature, we measured P Y – H Y at 300 K. As shown in Fig. 4d , P irreversibly changed under the weak field only during the first sweep even at 300 K. The difference between the first (red) and second (blue) profiles shows that the irreversible component of P Y amounted to 600 μ C m −2 at 300 K, as shown by the black line, which is almost comparable with or even larger than those measured at 4.2 K. Further, P steeply changed when the μ 0 H was between 12 and 14 T. Our P – H measurements at various temperatures revealed that this anomaly is smoothly connected with the one measured at low temperature when μ 0 H ~18 T ( Supplementary Fig. 2 and Supplementary Note 2 ) and, hence, can be interpreted as the magnetic transition to the canted antiferromagnetic state. Although our simple interpretation partly explains the observed change in the in-plane polarization, this domain model alone cannot explain the irreversible component measured at μ 0 H <10 T. According to this simple model, applying the H along the Y direction stabilized the Q 2 domain, which would have the largest component of P || Y . As shown in Fig. 4d , however, the initial point of the first sweep showed higher polarization than that of the second sweep, where we believe only the Q 2 domain existed. The origin for this additional P remains open at present. Judging from the magnetization and linear ME effect above 27 T (the red traces in Figs 2a and 3a ), the spin canting with the weak ferromagnetic moment of 0.1 μ B per Fe along the Z direction can induce P Y ~200 μ C m −2 . Possible emergence of weak ferromagnetic moment at the domain wall region [32] might contribute somewhat to this extra component. Further systematic study will be necessary to solve this mystery. Owing to the large electric polarization along the c axis, that is, the corresponding lattice distortion, spins in BiFeO 3 exhibit the cycloidal order. According to the generalized microscopic theory for anti-symmetric spin-dependent polarization [30] , [31] , this spin order involves parasitic spin-driven electric polarizations along with and also normal to the c axis. In BiFeO 3 , the latter coupling d YY is larger than the former one d ZY caused by the the spin current mechanism. This transverse component is confined to the magnetic domains and, hence, is easily controlled by H . The energy required for domain rotation can be estimated from the magnetization curve shown in Fig. 2b as ∫ BdM =1.18 × 10 3 J m −3 at 4.2 K. From this energy density, we can expect that transverse polarization of 600 μ C m −2 can be flopped by an electric field of 2 MV m −1 . This crude estimation reasonably agrees with the reported change in volume fraction of magnetic domains by electric field of 1.3 MV m −1 along the cubic axis [33] . Despite this small energy, the domain arrangement is preserved after removal of the H even at 300 K. These results indicate potential use of BiFeO 3 as a three-state non-volatile memory corresponding to the three Q vectors Q 1 , Q 2 and Q 3 . In conclusion, we studied the magnetic field dependence of the electric polarization in BiFeO 3 single crystals grown using the laser-diode heating floating-zone method. The electric polarization normal to the c axis showed prominent field-induced change. The irreversible low-field polarization was memorized by the field sweep. Such non-volatile memory effect was also observed even at 300 K, suggesting that the BiFeO 3 can be useful for novel memory devices. Experiments in high magnetic fields Pulsed magnetic fields up to 56 T were generated by using pulse magnets installed at the Institute for Solid State Physics at the University of Tokyo. The magnetization was measured using the induction method in pulsed fields. We used a commercial magnetometer (MPMS; Quantum Design) for the magnetization measurements up to 7 T, as shown in Fig. 2b . The field-induced changes in the electric polarization were calculated by numerically integrating the polarization currents [34] . To subtract the contribution of the voltage induced in the wiring, we averaged the signals measured during the positive and negative field sweeps ( Supplementary Fig. 3 and Supplementary Note 3 ). How to cite this article: Tokunaga, M. et al. Magnetic control of transverse electric polarization in BiFeO 3 . Nat. Commun. 6:5878 doi: 10.1038/ncomms6878 (2015).